Divergent synthesis of benzazepines and bridged polycycloalkanones via dearomative rearrangement 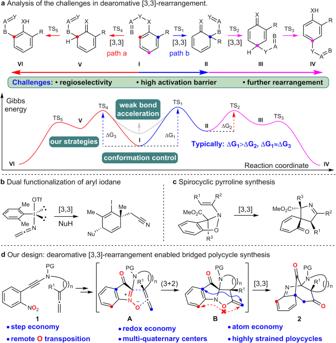Fig. 1: Dearomative [3,3]-rearrangement in efficient synthesis. aAnalysis of the challenges in dearomative [3,3]-rearrangement.bDual functionalization of aryl iodane.cSpirocyclic pyrroline synthesis.dOur design: dearomative [3,3]-rearrangement enabled bridged polycycle synthesis. PG = protective group. The dearomative functionalization of aromatic compounds represents a fascinating but challenging transformation, as it typically needs to overcome a great kinetic barrier. Here, a catalyst-free dearomative rearrangement of o -nitrophenyl alkyne is successfully established by leveraging the remote oxygen transposition and a weak N-O bond acceleration. This reaction features high atom-, step- and redox-economy, which provides a divergent entry to a series of biologically important benzazepines and bridged polycycloalkanones. The reaction is proposed to proceed through a tandem oxygen transfer cyclization/(3 + 2) cycloaddition/(homo-)hetero-Claisen rearrangement reaction. The resulting polycyclic system is richly decorated with transformable functionalities, such as carbonyl, imine and diene, which enables diversity-oriented synthesis of alkaloid-like polycyclic framework. The dearomative functionalization of aromatic compounds represents a fascinating transformation, which could rapidly build up stereocomplex 3-D alicyclic architectures with transformable C=C bonds from planar arenes in one step. Consequently, many successful approaches have been established during the last few decades [1] , [2] , [3] , [4] , [5] . From the perspective of arene substrates, most methods typically rely on low aromaticity arenes, such as phenol [6] , [7] , π-extended (hetero)arenes [8] , [9] , and hapto-coordinated arenes [10] . In terms of the thermodynamic profiles, highly active species such as cation [11] , carbene [12] , [13] , [14] , [15] , radical [16] , photoexcited intermediates [17] , [18] , and allyl organometallics; [19] , [20] were usually applied in order to compensate the enthalpic penalty in breaking an aromatic system. In this vein, catalytic asymmetric dearomatization has become a powerful method in achieving optically pure molecules from arenes [2] , [21] , [22] , [23] , [24] . Additionally, redox manipulation of the arene could also lead the loss of aromaticity, but stoichiometric strong oxidants [7] , [25] , [26] or reductants [27] , [28] , [29] were required in many cases. Strangely, in spite of these achievements, there are only a few reports of dearomative arene functionalization by leveraging an aromatic [3,3]-sigmatropic rearrangement strategy [5] , [30] , [31] , [32] , [33] , [34] , [35] , which proceed through a dearomative intermediate. Several inherent challenges might result in the scarcity of such a dearomative [3,3]-rearrangement (Fig. 1a ). Firstly, it is well-known that dearomatization processes have to overcome a prominent activation barrier (Fig. 1a , ΔG 1 and ΔG 3 ), which could not be sufficiently compensated from the enthalpy of sigma bond interchange during [3,3]-sigmatropic rearrangement. Secondly, the potential regioselectivity issues should be considered in developing such a reaction (Fig. 1a , paths a and b), so symmetrical or reactivity-differentiated substrates were usually applied [36] , [37] , [38] . Finally, the transiently formed dearomative intermediates are unstable and would easily collapse via rearomatization or consecutive [3,3]-sigmatropic rearrangement (Fig. 1a , product IV and VI ) [39] . Recently, several excellent studies aiming to address the activity issues were achieved by developing new catalytic model [8] , [32] or using energetic intermediates and substrates [37] , [38] , [40] , [41] . For example, Peng group disclosed a dearomative dual functionalization of aryl iodanes by integration a iodonio-Claisen rearrangement with a subsequent nucleophilic interception of the dearomative intermediate (Fig. 1b ) [38] . Anderson and coworkers reported a tandem of (3 + 2) cycloaddition and hetero-Claisen rearrangement for the dearomative synthesis of spirocyclic 1-pyrrolines by exploiting the activity of nitrones and arynes (Fig. 1c ) [40] . However, to the best of our knowledge, access to a bridged polycyclic system via dearomative [3,3]-sigmatropic rearrangement is still a yet unmet challenge. Inspired by these intriguing achievements and our successful experiences in dearomative Claisen rearrangement [42] , [43] , [44] , we intend to use the weak N-O bond (N-O: 53 kcal/mol vs C-O: 86 kcal/mol) as leverage to design the dearomative [3,3]-sigmatropic rearrangement, aiming for the synthesis of bridged alicyclic systems [45] . Fig. 1: Dearomative [3,3]-rearrangement in efficient synthesis. a Analysis of the challenges in dearomative [3,3]-rearrangement. b Dual functionalization of aryl iodane. c Spirocyclic pyrroline synthesis. d Our design: dearomative [3,3]-rearrangement enabled bridged polycycle synthesis. PG = protective group. Full size image In the past few decades, the (3 + 2) cycloadditions of nitrone have become a valid approach to assemble the N-O bond containing rings [45] , especially integrated with the alkyne chemistry [46] , [47] , [48] , [49] , [50] , [51] . For example, the nitroalkyne-based oxygen transfer could efficiently generate the nitrone, which can then be intercepted by an intermolecular alkene to give a polycyclic system [48] , [49] , [50] . Similarly, we surmised that an in-situ generated nitrone bearing a well-situated allene would undergo selective cycloaddition and the conformation of the newly formed ring would ensure the consequent dearomative sigmatropic rearrangement occurring selectively to give a stereochemically and functionally rich bridged polycyclic system (Fig. 1d ). In this work, we disclose a catalyst-free dearomative [3,3]-rearrangement of o -nitrophenyl alkyne for the divergent synthesis of benzazepines and bridged polycycloalkanones via remote oxygen transposition (over 11 atoms). This reaction features high atom-, step- and redox-economy. In addition, the resulting polycyclic system is constituted by four rings, two bridge-head quaternary centers, and transformable functionalities of cyclohexadiene and cyclodiketone, which enables the diversity-oriented synthesis of alkaloid-like fused polycyclic frameworks. Serendipitous discovery and rationalization To verify our hypothesis, we set out the investigation with the easily available ynamide 1a as model substrate. Surprisingly, under thermolysis conditions, the desired bridged cycloalkanone was not detected, but an unknown compound with one carbon atom less (identified by NMR) was isolated in 81% yield (Fig. 2a , entry 3). The temperature has great impact on the reaction yields (Fig. 2a ). The structure was tentatively assigned to benzazepine 2a by analysing of the NMR spectra, which was further confirmed later by the X-ray crystal diffraction analysis of the analogue 2k (Fig. 3 ). The formation of benzazepine 2a can be rationalized as shown in Fig. 2b . The thermal-triggered intramolecular oxygen transfer [48] , [49] , [50] of 1a initially gave the nitrone III (Fig. 2b ), which could be effectively trapped by the tethered allene with complete diastereoselectivity. The resulting (3 + 2) cycloaddition adduct IV then underwent the dearomative [3,3]-sigmatropic rearrangement to afford the bridged cycloalkanone 2a’ , one molecule of carbon monoxide (CO) was further extruded through a cheletropic decarbonylation reaction (retro (4 + 1) reaction for simplicity) [52] , [53] , [54] , [55] , [56] to regenerate the benzene ring and followed by isomerization to give the thermodynamically favourable product 2a . It is noteworthy that the CO gas could be detected by GC analysis of the gas in the reaction flask (see SI for details). The extrusion of CO was presumably due to the high tendency of rearomatization and high ring strain of the intermediate 2a’ . Fig. 2: Reaction optimization and mechanistic rationalization. a Serendipitous discovery and reaction optimization. b Rationalization of the mechanism of the serendipitously observed 2a . c Selected representative drug molecules and important bioactive benzazepine scaffolds. Ts = p -toluenesulfonyl. Bn = benzyl. Full size image Fig. 3: Evaluation of scope of benzazepines a . a Reaction conditions: The solution of 1 in THF (0.03 M) was stirred under N 2 atmosphere at 90 o C for 6 h. b Heating the resulting filtrate of 1 after the ynamide formation. PG = protective group. Ts = p -toluenesulfonyl. Ms = methanesulfonyl. Full size image Scope of the benzazepines Encouraged by our initial discovery and the important bioactivity of benzazepines (Fig. 2c ) [57] , [58] , [59] , [60] , we then started to test the generality of this reaction under the optimized conditions (Fig. 2a , entry 3). As shown in Fig. 3 , the electronic nature of the arene has little influence on the formation of the benzazepines ( 2a-n ) except the methylenedioxy-substituted product 2i . Both electron-rich and electron-deficient benzazepines were isolated in similar yields (about 70%). It is worth noting that the sterically hindered product 2n could obtained in 59% yield as well. Interestingly, the otherwise difficult to access pyridine-fused azepine 2o was also achieved in moderate yield (52%). In addition, the internal allene tethered substrates were subjected to the standard reaction conditions as well, giving the desired benzazepines 2p and 2q in 47% and 75% yield, respectively. Finally, the piperidine-fused benzazepine 2r and methylsulfonyl-protected benzazepine 2 s could also be obtained in satisfactory yields. Having realized the formation of benzazepines, we wondered if the originally desired bridged polycyclic system could be accessed through the stabilization of the transient dearomatized intermediate via minimization of ring strain (Fig. 4 ). As the ring strain will drastically reduce with the increasing of ring size, therefore, we tried to extend the [3.2.1]-bridged system to a [n.2.1]-bridged one (n > 3). Inspired by the homo-Nazarov cyclization reaction [61] , [62] , [63] and also the mechanistic fact that the [3,3]-sigmatropic rearrangement might involve a diradical species [39] , replacing one C=C bond of the allene with a cyclopropane moiety [64] may enable a homo-Claisen rearrangement and lead to the desired [4.2.1]-bridged polycyclic product 4 without CO extrusion. It is worthy to note that a radical mediated Brandi rearrangement [65] , [66] , [67] , in addition to the competitive retro (4 + 1) addition reaction, might be involved as well, which further complicated the reaction system. Fig. 4: Minimization of ring strain in achieving bridged polyclcloalkanone. The homo-hetero-Claisen rearrangement postulation inspired by mechanistic insight of Claisen rearrangement and the homo-Nazarov cyclization. PG = protective group. Full size image Scope of the bridged polyclcloalkanones With these considerations in mind, we then set out to validate the feasibility of such hypothesis. Fortunately, when nitroalkyne 3a with a tailored methylenecyclopropane was applied as substrate, the envisioned dearomative bridged polycyclic product 4a was obtained in 74% yield, which was unambiguously confirmed by X-ray crystal diffraction analysis (Fig. 5 ). To the best of our knowledge, it is the first homo-hetero-Claisen rearrangement reaction. It is also noteworthy that in this cascade process the two oxygen atoms of the nitro group were transferred over 4 and 11 atoms, giving two transformable ketone functionalities in a redox-neutral manner. In line with our previous observation, the electronic properties and substituted patterns of the arene have little effect on the reaction performance ( 4a - p , 60-81%). For example, the nitrobenzenes with -CO 2 Me or -OMe group at the meta-position could deliver the desired products 4b and 4 h in excellent yields. In addition, the methylenedioxy substituted product 4j could be obtained in 76% yield, which is in stark contrast to that of 2i (22%). Notably the formation of 4o needed a slightly elevated temperature and prolonged reaction time (80 o C, 36 h), which might be attributed to the steric hindrance. The practicability of the naphthalene and pyridine-based substrates were also tested to give the corresponding products 4q and 4r in satisfactory yields. The reaction was highly sensitive to the size of R 2 as the yields decreased sharply when the group R 2 was replaced by ethyl and phenyl, furnishing the corresponding products 4 s and 4t in only 36% and 21% yield, respectively. When ynamide with a shorter tether were used as substrates, the desired products decomposed quickly upon chromatography isolation on silica gel. Fortunately, these in situ generated polycyclic diketones could be selectively reduced to the corresponding alcohols 4 u’ and 4 v’ in 68% and 45% yield, respectively. It is worthy to mention that the dimethyl amine substituted product 4 v could be observed by NMR in 62% yield, but it was sensitive to silica gel and transformed to the ring fragmentation product 4w’ in 58% yield. In addition, methylsulfonyl- and o -nitrobenzenesufonyl protected polycyclic product 4x and 4 y could also be obtained in good yield. In sharp contrast to the sulfonyl protected counterparts, the carbamate protected substrate 3z required more forcing conditions (100 o C for 120 h), delivering the desired bridged adduct 4z in 62% yield with the thermolabile tert-butoxycarbamate moiety survived. Interestingly, when the cyclobutene-containing substrate was tested, however, only the (3 + 2) adduct 4aa’ was isolated in excellent yield, which couldn’t be further transferred to the desired bridged cyclic product even elevating the reaction temperature to 200 o C, which indicated that the weak N-O bond is thermally stable and the cyclopropane is critical for the following rearrangement. Fig. 5: Evaluation of scope of benzazepines a . a Reaction conditions: The solution of 3 in THF (0.03 M) was stirred under N 2 atmosphere at 75 o C for 12 h; b Heating the resulting filtrate of 3 after the ynamide formation; c 80 °C for 36 h; d NaBH 4 (3 eq) and 0.5 mL MeOH were added when the rearrangement reaction mixture cooling to room temperature, then stirred for another 1 h. Note: these imine-containing bridged skeletons are quite stable, without obvious decomposition when placed under ambient atmosphere and temperature for more than 2 months. PG = protective group. Ts = p -toluenesulfonyl. Ms = methanesulfonyl. Ns = 2-nitrobenzenesulfonyl. Boc = t-butoxycarbonyl. THF = tetrahydrofuran. Full size image The compatibility of other type substrates To further explore the reaction scope, other type of nitroalkynes were tested as substrates as well (Fig. 6 ). Unexpectedly, a low conversion was achieved when the alkynyl thioethers were tested as the substrates under the standard conditions, which was in striking contrast to Verniest’s results [48] . When the reaction temperature was increased from 75 o C to 120 o C, the thioether 3ab exclusively afforded the endo -cycloaddition adduct 4ab’ rather than the desired bridged dione 4ab . Such selectivity inversion indicated that the steric repulsion between the Ts group and cyclopropane moiety is critical in ensuring the exo -cycloaddition and the subsequent rearrangement processes. We further envisioned that a shorter tether might alter the reaction selectivity in favoring exo -cycloaddition as the ring tension would increase dramatically for the endo -selectivity. Surprisingly, the thioether 3ac with one less carbon atom delivered a bridged-carbonyl group transposed product 4ac’ without observing 4ab’ -like endo -adduct. In addition, the allene thioether 1t was also examined, which gave the benzazepines 2t and 2t’ , which might arise from an asynchronous heterolysis [54] of transient bridged product 4t . In addition to the substrates with heteroatom-modified and electronically biased carbon-carbon triple bond (ynamide and thioalkyne), the nitroalkynes 3ad and 3ae with carbon atom-capped carbon-carbon triple bond were explored as well. Interestingly, the substrate 3ad could transfer to 4ad’ and 4ad” upon exposure to air at room temperature over a period about two months. The structure of 4ad” was unambiguous validated by X-ray diffraction analysis. However, under thermal conditions, the substrate decomposed dramatically (>150 °C) with only trace amount of the desired products were observed by NMR analysis of the reaction mixture. The formation of the endo -adduct 4ad’ confirmed again the steric effect is very important, which is in line with the observation in 3ab . For the propiolamide 3a , the reaction is sluggish under heating conditions (150 o C for 8 h). A cooperative strategy by combined the gold catalysis [49] , [50] and the thermolysis process was also applied. However, we could not detect the desired product 4ae , but with its descendant 4ae’ being isolated in 7% yield, which might proceed through the intermediate 4ae-Int with the assistance of gold coordination and nucleophilic chloride. Fig. 6: Test the compatibility of other type substrates. a The solution of 3 in toluene (0.03 M) was stirred under N 2 atmosphere at 110 or 120 o C for 12 h; b The viscous oil 3ad (50 mg) in a 25 mL round bottom flask with a stopper was stood at room temperature for 60 days; c To the solution of 3ae in PhMe (0.03 M) was added PicAuCl 2 (0.2 eq) under nitrogen atmosphere, then stirred at 100 °C for 12 h. n.d. means not detected. Pic = 2-pyridinecarboxylate. Ts = p -toluenesulfonyl. Bn = benzyl. Full size image Mechanistic study To better understand the reaction mechanism, several control reactions were then conducted. Intuitively, we think that a loose radical pair involved pathway [39] might be more feasible as tremendous transannular strain will built-up in achieving a synchronic [3,3]-sigmatropic rearrangement transition state. Therefore, the cyclopropane substituted substrate 1 u was applied to probe the intermediacy of such radical pair. However, no ring opening products, such as 2 u’ , were detected, but with the normal benzazepine 2 u being isolated in good yield (Fig. 7 , Eq. 1). In addition, the attempt to intercept or terminate the envisioned radical species with TEMPO and Et 3 SiH also failed (Eq. 2). Finally, 3a was conducted on a gram scale in order to detect the potential Brandi cyclization product 4a’ , which typically proceeded through a radical pathway [65] , [66] , [67] . Similarly, the normal rearrangement product 4a was obtained in 65% yield, while no desired Brandi cyclization product 4a’ was isolated even in trace amount (Eq. 3). These results indicated that the postulated radical pair either reluctant to be perturbated from outside or not existed. Introducing 4 equivalents of H 2 18 O to the reaction system has no effect on the reaction outcome (72%), which further confirmed its robustness. 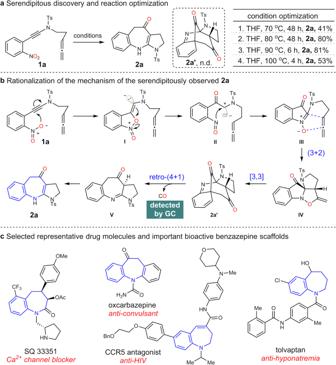Fig. 2: Reaction optimization and mechanistic rationalization. aSerendipitous discovery and reaction optimization.bRationalization of the mechanism of the serendipitously observed2a.cSelected representative drug molecules and important bioactive benzazepine scaffolds. Ts =p-toluenesulfonyl. Bn = benzyl. The HRMS and 13 C-NMR of resulting product revealed that no 18 O was incorporated (Eq. 4), which corroborated that the carbonyl groups came from the transposition of oxygen of nitroxide rather than external water. In addition, the reaction profiles were monitored by in situ IR spectroscopy, which characterized by the stretching vibration absorption of two carbonyl groups at 1720 cm −1 and 1775 cm −1 , while no obvious absorption of intermediates were accumulated throughout, indicating their metastable character. Taken together, we are preferred more to a concerted but asynchronous [3,3]-sigmatropic rearrangement process wherein the N-O cleavage more advanced to relieve the incoming transannular strain. Fig. 7: Mechanistic investigation and gram-scale synthesis. a Control experiments: The Eqs. 1 and 2 indicate that no radical is involved in the (homo-)hetero-Claisen rearrangement. Eq. 3 is robust and radical mediated Brandi cyclization occurred, which imply the absence of radical species in the homo-hetero-Claisen rearrangement. b Investigation of the cascade reaction profiles by the in situ IR spectroscopy. THF = tetrahydrofuran. Ts = p -toluenesulfonyl. Full size image With the bridged polycyclic compounds in hand, efforts to demonstrate the synthetic utility of them were then conducted (Fig. 8 ). The stereochemically and functionally rich polycyclic systems could be successfully converted into a series of alkaloid-like frameworks ( 5-14 ) by using very simple and practical procedures (6-7 steps in total from the commercially available starting material). Taking 4a as an example, the two carbonyl groups could be selectively differentiated under the Wittig reaction conditions to give the olefin 5 in 51% yield. Interestingly, the reduction of 4a with sodium borohydride gave alcohol 6 in 2.2:1 dr, while under the otherwise identical conditions except nickel chloride, a cage product 7 was obtained in high yield, which might arise from the selective ketone reduction, C=C bond hydration and acetalation processes. In addition, under the Luche reduction conditions, a similar cage product 8 with one C=C reserved was furnished in excellent yield. Under more forcing conditions, another cage compound 9 with the bridged carbonyl group being reduced could be isolated in 80% yield. These complex architectures were confirmed by the X-ray analysis ( 7 , 8 and 9 ). In addition, selective reduction of one C=C bond of the cyclohexadiene could also be achieved with the Hantzsch ester as hydride donor, giving the product 10 in 91% yield. Epoxidation of the less sterically hindered C=C bond was feasible, but accompanied by the oxidation of imine motif. The stereochemistry of the epoxide 11 was also established by X-ray diffraction analysis. Reducing the loading of m- CPBA would selectively produce the kinetic product 12 in good yield. Under basic conditions in the presence of silica gel, a ring fragmentation product 13 was obtained in moderate yield. Exposing 13 to the acid condition led to a bis-spiral system 14 , which was also confirmed by X-ray diffraction analysis. Interestingly, the spiral indolone 14 could also be obtained in 77% yield by treating 4a with trifluoroacetic acid at 90 o C for 6 h. The Boc-protected product 4z was labile to acidic condition, with the bridged architecture collapse to a planar molecule 15 at room temperature in quantitative yield. Finally, further transformation of benzazepine 2a was conducted to demonstrate its versatile capacity in diversification modification the benzazepine skeleton. As many of the vaptan class of drugs contain a N-linked benzoyl moiety [57] , [68] , [69] , the benzoylation product 16 was synthesized preferentially. Interestingly, the peripheral pyrrole unit could shift to another position under refluxing acidic environment to give 17 in good yield. Fig. 8: Late-stage diversification of 4a and 2a. Selective olefination and reduction of the dione to give 5 and 6 . Reductive acetalation companied with entirely reduction of the diene to afford the cage product 7 . Luche reduction conditions could also produce the cage product 8 with the cyclohexadiene partially hydrogenated. The bridged carbonyl group could be reduced with lithium aluminium hydride to furnish 9 . One C = C double bond of the cyclohexadiene was selectively reduced by Hantzsch ester to provide 10 . Epoxidation product 11 was obtained with m -CPBA. Kinetically oxidation of the imine moiety to give nitrone 12 . Retro Michael addition to give the fragmentation oxindole 13 , which could transform to the spiral dione 14 . Under the acidic deprotection conditions the three-dimensional architecture of 4z collapsed entirely to form a unique [6-6-5-6] tetracyclic architecture 15 . Furthermore, the benzoyl functionality could be easily installed on free nitrogen atom of 2a to give product 16 . Interestingly, compound 2a has been structurally reorganized into a [6-7-5] tricyclic architecture 17 by refluxing in TsOH/methanol solution. m -CPBA = m -chloroperoxybenzoic acid. TEA = triethylamine. TFA = trifluoroacetic Acid. DMAP = 4-(dimethylamino)pyridine. Ms = methylsulfonyl. Ts = p -toluenesulfonyl. 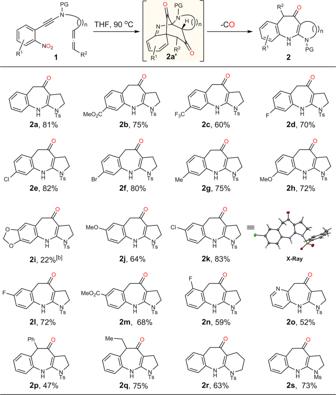Fig. 3: Evaluation of scope of benzazepinesa. aReaction conditions: The solution of1in THF (0.03 M) was stirred under N2atmosphere at 90oC for 6 h.bHeating the resulting filtrate of1after the ynamide formation. PG = protective group. Ts =p-toluenesulfonyl. Ms = methanesulfonyl. Boc = t -butoxycarbonyl. NaBH 4 = sodium borohydride. LiAlH 4 = lithium aluminum hydride. Full size image The antiviral activity The approved anti-HIV drug, nevirapine, is a benzazepine analogue. Therefore, we firstly evaluated the chemotype 2 compounds (with benzazepine scaffold) using as nevirapine the positive control. As results, the chemotype 2 compounds only showed modest anti-HIV activity in SupT1 cells at 10 µM concentration (Table S3 ). To explore whether these unique architectures of 4 and its derivatives could serve as potential bioactive agents with novel core structure, we performed chemical structure similarity search in therapeutic target database (TTD) using the core structure of this series compound as the template, and four compounds were obtained with the Tanimoto similarity more than 0.7. The most similar compound Spiro[pyrrolidine-2,2-adamantane] (Tanimoto similarity was 0.745) was identified with the antiviral activity against influenza A virus (IAV) and the human immunodeficiency virus type 1 (HIV-1) and type 2 (HIV-2). Therefore, we explored the bioactivity of these compounds via testing the antiviral activity of IAV and HIV-1. As results, preliminary anti-HIV-1 assay indicated that compound 13 displayed the best anti-HIV effect with 97% reduction of VSV-G-pseudotyped HIV-1 virus in SupT1 cells at 10 µM concentration (Table S4 ). Further testing showed that 13 inhibited HIV-1 in a dose dependent manner (EC 50 = 4.24 µM, Fig. 9a ). However, the antiviral potency was measured in a Luc reporter assay which could not separate inhibition from the cytotoxicity. Therefore, the observed Luc reduction shown in Fig. 9a may largely reflect the cytotoxicity of 13 in SupT1 cell lines (CC 50 = 8.22 µM, Fig. 9b ). As for the antiviral activity against IAV, most of the compounds under preliminary test exhibited anti-IAV activity in 293T-GLUC cell at 10 µM concentration (Table S5 ), and 4a displayed the best anti-IAV effect with 92% reduction of IAV virus. Further activity inspection indicated 4a could inhibit the growth of IAV virus in dose dependent manner with the EC 50 of 7.73 µM (Fig. 9c ). Importantly, 4a exhibited low cytotoxicity (not showing cytotoxicity up to 50 µM) for 293T-GLUC cell (Fig. 9d ), suggesting that the observed antiviral effect was not due to cytotoxicity. Taken together, this series compound would become a type of promising anti-virus agents with brand new scaffold. Fig. 9: The antiviral activity. a 13 inhibited the growth of HIV-1 virus in dose dependent manner in SupT1 cell; b 13 exhibited moderate cytotoxicity with CC 50 of 8.22 µM for SupT1 cell; c 4a inhibited the growth of IAV virus in dose dependent manner in 293T-GLUC cell; d 4a exhibited low cytotoxicity for 293T-GLUC cell. ( n = 3). Bar = mean. Error bars = ±SEM. Data are from at least three independent experiments and evaluated via Prism (version 5.01, GraphPad Software, San Diego, CA, USA). Full size image In summary, we disclosed a dearomative rearrangement, which enable divergent accesses to a series of unique benzazepines and bridged polycycloalkanones in a redox-neutral, step- and atom-economic manner. The reaction was proposed to proceed through a tandem oxygen transfer cyclization/(3 + 2) cycloaddition/(homo-)hetero-Claisen rearrangement reaction, wherein an oxygen atom was eventually transposed over 11 atoms. The resulting bridged polycycloalkanones could be successfully converted into several alkaloid-like frameworks via late-stage diversification. The preliminary bioactivity investigation indicated that these unique bridged frameworks hold great potential to be a type of promising anti-virus agents with brand new scaffold. 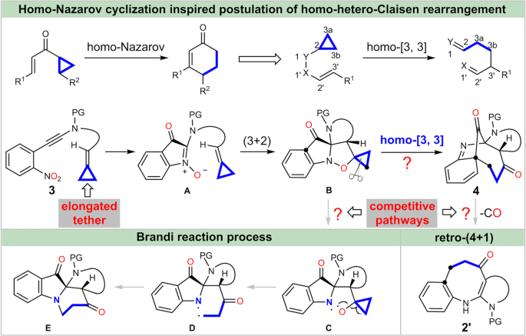Fig. 4: Minimization of ring strain in achieving bridged polyclcloalkanone. The homo-hetero-Claisen rearrangement postulation inspired by mechanistic insight of Claisen rearrangement and the homo-Nazarov cyclization. PG = protective group. 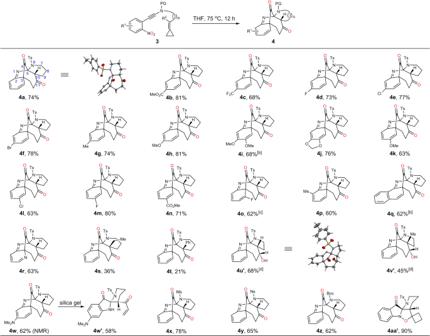Fig. 5: Evaluation of scope of benzazepinesa. aReaction conditions: The solution of3in THF (0.03 M) was stirred under N2atmosphere at 75oC for 12 h;bHeating the resulting filtrate of3after the ynamide formation;c80 °C for 36 h;dNaBH4(3 eq) and 0.5 mL MeOH were added when the rearrangement reaction mixture cooling to room temperature, then stirred for another 1 h. Note: these imine-containing bridged skeletons are quite stable, without obvious decomposition when placed under ambient atmosphere and temperature for more than 2 months. PG = protective group. Ts =p-toluenesulfonyl. Ms = methanesulfonyl. Ns = 2-nitrobenzenesulfonyl. Boc = t-butoxycarbonyl. THF = tetrahydrofuran. General procedure for the synthesis of benzazepines and bridged polycycloalkanones A dried 25 mL Schlenk tube was flushed with nitrogen three times. The solution of 1 (or 3 ) in the THF (0.03 M) was added to the tube under nitrogen atmosphere. 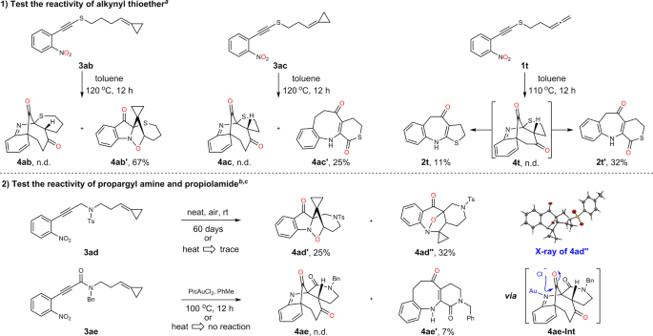Fig. 6: Test the compatibility of other type substrates. aThe solution of3in toluene (0.03 M) was stirred under N2atmosphere at 110 or 120oC for 12 h;bThe viscous oil3ad(50 mg) in a 25 mL round bottom flask with a stopper was stood at room temperature for 60 days;cTo the solution of3aein PhMe (0.03 M) was added PicAuCl2(0.2 eq) under nitrogen atmosphere, then stirred at 100 °C for 12 h. n.d. means not detected. Pic = 2-pyridinecarboxylate. Ts =p-toluenesulfonyl. Bn = benzyl. The resulting mixture was put in a 90 °C (or 75 °C for 3 ) oil bath and stirred for 6 h (or 12 h for 3 ). After cooled to room temperature, the mixture was transferred to a 25 mL round bottom flask and evaporated under reduced pressure. The residue was purified by column chromatography on silica gel (petroleum ether/EtOAc as eluent) to give desired cyclization product 2 (or 4 ). 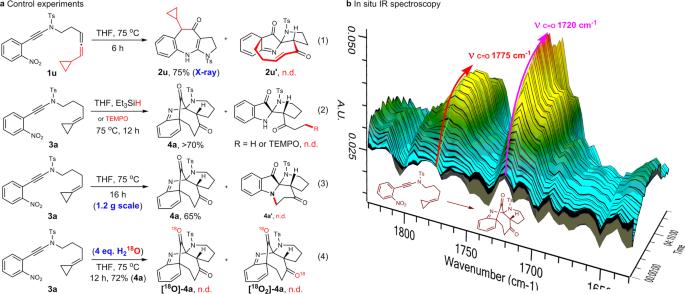Fig. 7: Mechanistic investigation and gram-scale synthesis. aControl experiments: The Eqs. 1 and 2 indicate that no radical is involved in the (homo-)hetero-Claisen rearrangement. Eq. 3 is robust and radical mediated Brandi cyclization occurred, which imply the absence of radical species in the homo-hetero-Claisen rearrangement.bInvestigation of the cascade reaction profiles by the in situ IR spectroscopy. THF = tetrahydrofuran. Ts =p-toluenesulfonyl. 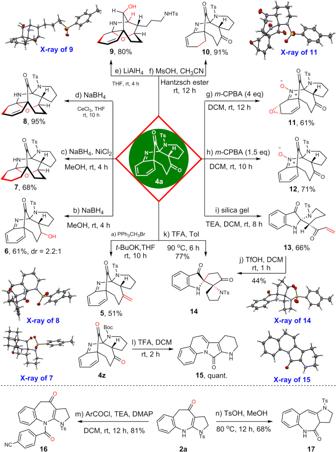Fig. 8: Late-stage diversification of 4a and 2a. Selective olefination and reduction of the dione to give5and6. Reductive acetalation companied with entirely reduction of the diene to afford the cage product7. Luche reduction conditions could also produce the cage product8with the cyclohexadiene partially hydrogenated. The bridged carbonyl group could be reduced with lithium aluminium hydride to furnish9. One C = C double bond of the cyclohexadiene was selectively reduced by Hantzsch ester to provide10. Epoxidation product11was obtained withm-CPBA. Kinetically oxidation of the imine moiety to give nitrone12. Retro Michael addition to give the fragmentation oxindole13, which could transform to the spiral dione14. Under the acidic deprotection conditions the three-dimensional architecture of4zcollapsed entirely to form a unique [6-6-5-6] tetracyclic architecture15. Furthermore, the benzoyl functionality could be easily installed on free nitrogen atom of2ato give product16. Interestingly, compound2ahas been structurally reorganized into a [6-7-5] tricyclic architecture17by refluxing in TsOH/methanol solution.m-CPBA =m-chloroperoxybenzoic acid. TEA = triethylamine. TFA = trifluoroacetic Acid. DMAP = 4-(dimethylamino)pyridine. Ms = methylsulfonyl. Ts =p-toluenesulfonyl. Boc =t-butoxycarbonyl. NaBH4= sodium borohydride. LiAlH4= lithium aluminum hydride. 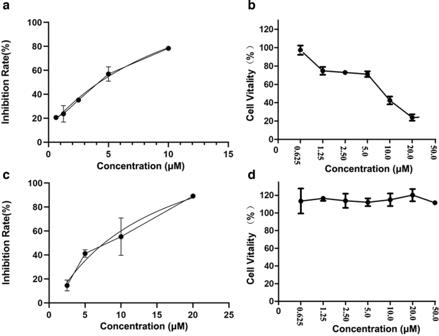Fig. 9: The antiviral activity. a 13inhibited the growth of HIV-1 virus in dose dependent manner in SupT1 cell;b 13exhibited moderate cytotoxicity with CC50of 8.22 µM for SupT1 cell;c 4ainhibited the growth of IAV virus in dose dependent manner in 293T-GLUC cell;d 4aexhibited low cytotoxicity for 293T-GLUC cell. (n= 3). Bar = mean. Error bars = ±SEM. Data are from at least three independent experiments and evaluated via Prism (version 5.01, GraphPad Software, San Diego, CA, USA). Reporting summary Further information on research design is available in the Nature Research Reporting Summary linked to this article.